Direct measurement of the absolute absorption spectrum of individual semiconducting single-wall carbon nanotubes The optical properties of single-wall carbon nanotubes are very promising for developing novel opto-electronic components and sensors with applications in many fields. Despite numerous studies performed using photoluminescence or Raman and Rayleigh scattering, knowledge of their optical response is still partial. Here we determine using spatial modulation spectroscopy, over a broad optical spectral range, the spectrum and amplitude of the absorption cross-section of individual semiconducting single-wall carbon nanotubes. These quantitative measurements permit determination of the oscillator strength of the different excitonic resonances and their dependencies on the excitonic transition and type of semiconducting nanotube. A non-resonant background is also identified and its cross-section comparable to the ideal graphene optical absorbance. Furthermore, investigation of the same single-wall nanotube either free standing or lying on a substrate shows large broadening of the excitonic resonances with increase of oscillator strength, as well as stark weakening of polarization-dependent antenna effects, due to nanotube–substrate interaction. For nanometric size objects, such as single-wall carbon nanotubes (SWNTs), the dominant interaction with light is due to their optical absorption. Understanding and quantitative characterization of the absorption processes and of their modification by the SWNT environment (for example, free-standing or substrate-deposited SWNTs) are crucial for their applications and, more generally, for fundamental comprehension of light–matter interaction in quasi one-dimensional nanomaterials [1] , [2] , [3] , [4] . Their precise investigation is made difficult by the large heterogeneities of the carbon nanotube (CNT) structural parameters in most synthesized CNT ensembles, leading to measurement of mean properties. This can be avoided by performing optical investigations at the individual nanotube level. Such approach has been increasingly developed during the last years, yielding optical imaging of individual CNTs and information on their excitonic resonant energies and linewidths [5] , [6] , [7] , [8] , [9] , [10] , [11] , [12] , [13] , [14] , [15] . No quantitative determination of the amplitude of the absorption cross-section was obtained, except at specific wavelengths using luminescence, thermal or Rayleigh scattering techniques [9] , [14] , [16] , [17] . The key process of light absorption was however only indirectly addressed, which is probably at the origin of the large dispersion of the indirectly estimated cross-sections found in the literature. A major experimental challenge is thus to directly analyse the absorption of a SWNT, quantitatively and over a large spectral range. Very recently, a variant of the spatial modulation spectroscopy (SMS) technique, initially developed to quantitatively study the optical response of single metal nanoparticles [18] , [19] , has been successfully applied to the investigation of individual SWNTs on a substrate [15] . As compared with other optical techniques, SMS has the key advantage of being sensitive to the optical extinction of the studied nano-object and to directly measure its absolute extinction cross-section. In the case of SWNTs, extinction being dominated by absorption, the value of the absorption cross-section of deposited CNTs was thus determined at a few specific laser wavelengths [15] , [20] . In this work, we extend this method to investigate the absolute polarized absorption cross-section of individual suspended or deposited SWNTs over the full optical range. The optical spectral features (absorption peaks, spectral widths, amplitudes and oscillator strengths, and polarization anisotropy) of the different excitonic transitions in the visible–near-infrared range, as well as the non-resonant absorption background, are precisely determined and discussed for different SWNTs identified (size and chirality) by correlation with Raman spectroscopy. Furthermore, the impact of environment is directly evidenced by measuring the absorption cross-section spectra of the same SWNT free standing (suspended part over a trench) or deposited (supported part on a silicon substrate). Absolute absorption spectroscopy by spatial modulation Ultra-long CNTs were grown by chemical vapour deposition (CVD) on home-made silica on silicon (SiO 2 /Si) substrates presenting 20-μm wide trenches ( Fig. 1a and Methods). Individual SWNTs crossing a trench were investigated, permitting to determine their optical absorption spectra either in free-standing conditions ( Fig. 2a , Fig. 3a and Supplementary Fig. S1a,d ) or in interaction with the substrate ( Fig. 3d ), using SMS in transmission or in reflection (R-SMS, the substrate being opaque), respectively. They were individually characterized before and after optical absorption studies using resonant Raman spectroscopy (see Methods for details). Their diameters, d (nm), were extracted from the frequencies of their radial breathing modes (RBMs) using the relation ω RBM (cm −1 )=204/ d +27 for suspended nanotubes [21] , [22] . Their chiral indices were subsequently identified by comparing the optical resonances with the spectral position and spacing of the different excitonic transitions predicted by Kataura plots [23] , [24] , [25] (for more details see Supplementary Note 1 and Supplementary Table S1 ). 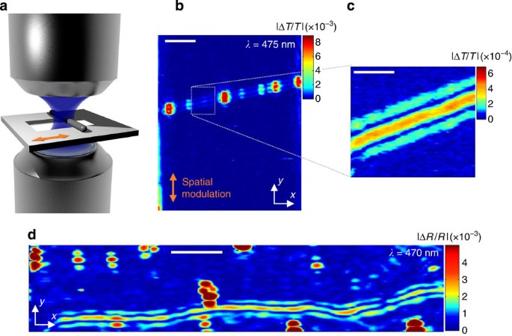Figure 1: Absorption-based imaging of SWNTs. (a) Sketch of the SMS technique showing the double microscope system and the sample. Its position is periodically modulated at frequencyf(orange arrow) and the transmitted beam power is synchronously detected at 2f. (b) Transmission SMS image, |ΔT/T(x,y)|, of a region of the trench showing the free-standing (22,6) individual semiconducting SWNT. (c) Zoom on a clean section of this nanotube. (d) Reflective R-SMS image, |ΔR/R(x,y)|, showing the substrate-supported part of the (14,13) semiconducting SWNT. Red spots in the optical images come from small dust particles. Scale bars, 3 μm (b); 1 μm (c); and 3 μm (d). Figure 1: Absorption-based imaging of SWNTs. ( a ) Sketch of the SMS technique showing the double microscope system and the sample. Its position is periodically modulated at frequency f (orange arrow) and the transmitted beam power is synchronously detected at 2 f . ( b ) Transmission SMS image, |Δ T / T ( x , y )|, of a region of the trench showing the free-standing (22,6) individual semiconducting SWNT. ( c ) Zoom on a clean section of this nanotube. ( d ) Reflective R-SMS image, |Δ R / R ( x , y )|, showing the substrate-supported part of the (14,13) semiconducting SWNT. Red spots in the optical images come from small dust particles. Scale bars, 3 μm ( b ); 1 μm ( c ); and 3 μm ( d ). 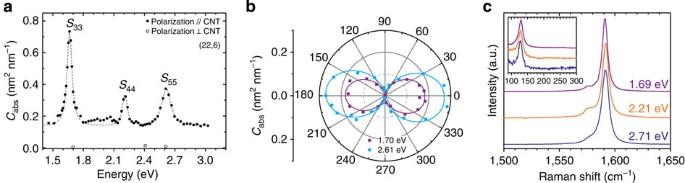Figure 2: Absorption and Raman spectroscopy of a free-standing individual SWNT. Results are presented for the (22,6) semiconducting SWNT. (a) Absolute absorption cross-section spectrum for incident light parallel (full dots) and perpendicular (open dots) to the nanotube. The dashed line is the result of the fit detailed in the main text. (b) Light polarization-dependent absorption cross-section for two laser excitation energies. The experimental data (symbols) are fitted by the function,θ=0 being the direction parallel to the nanotube axis. (c) Raman spectra showing the tangential modes and RBM (inset) measured with three different excitation energies labelled on the figure close to absorption peaks. Full size image Figure 2: Absorption and Raman spectroscopy of a free-standing individual SWNT. Results are presented for the (22,6) semiconducting SWNT. ( a ) Absolute absorption cross-section spectrum for incident light parallel (full dots) and perpendicular (open dots) to the nanotube. The dashed line is the result of the fit detailed in the main text. ( b ) Light polarization-dependent absorption cross-section for two laser excitation energies. The experimental data (symbols) are fitted by the function , θ =0 being the direction parallel to the nanotube axis. ( c ) Raman spectra showing the tangential modes and RBM (inset) measured with three different excitation energies labelled on the figure close to absorption peaks. 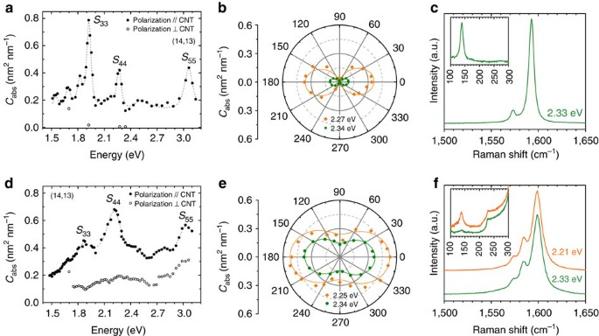Figure 3: Environment-dependent absorption and Raman scattering. The optical properties of the same (14,13) individual SWNT are investigated at both its freely suspended section (top panels) and its extremities supported on the silicon substrate (bottom panels). (a,d) Broadband absorption spectra, (b,e) light polarization-dependent absorption cross-sections (the polarization-dependent data are fitted by,θ=0 being the direction parallel to the nanotube axis) and (c,f) Raman spectra (with excitation energies labeled on the figure) are measured in the two situations. Full size image Figure 3: Environment-dependent absorption and Raman scattering. The optical properties of the same (14,13) individual SWNT are investigated at both its freely suspended section (top panels) and its extremities supported on the silicon substrate (bottom panels). ( a , d ) Broadband absorption spectra, ( b , e ) light polarization-dependent absorption cross-sections (the polarization-dependent data are fitted by , θ =0 being the direction parallel to the nanotube axis) and ( c , f ) Raman spectra (with excitation energies labeled on the figure) are measured in the two situations. Full size image The SMS method is based on modulating the position of a single nano-object placed under a tightly focused polarized light beam and detecting the induced modulation of the transmitted or reflected light energy. The experimental setup uses a double microscope system focusing and collecting the light close to diffraction limit with two high-numerical aperture × 100 objectives ( Fig. 1a ). The sample is fixed on a linear piezo-actuator, which permits fast spatial modulation of its position in the y direction at frequency f . An x – y positioning stage allows rastering of the sample with subnanometre precision. The modulated part of the transmitted, Δ T / T , or reflected Δ R / R (collected by the focusing objective) light at frequency 2 f is detected with a photodiode and a lock-in amplifier. In both cases, it directly provides the absolute absorption cross-section per unit length, C abs , of the studied nanotube at the incident light wavelength. More details concerning SMS and R-SMS, as well as the positioning and orientation of CNTs, are available elsewhere (see also Methods) [15] , [18] . Measurements of C abs spectra were performed for incident wavelength λ tunable in the 400 nm–850 nm range (that is, photon energies E ranging from 1.45 to 3.1 eV), provided either by a femtosecond Ti:Sapphire laser ( λ ranging from 700 to 1,000 nm), a visible optical parametric oscillator ( λ from 500 to 700 nm) or by second harmonic generation in a non-linear crystal ( λ from 400 to 500 nm). In all cases, the light beam is polarization-controlled and its spectral linewidth characterized (Gaussian intensity profile with a full-width at half-maximum (FWHM) ~14, 18 and 24 meV for the near-infrared, green and blue part of the spectra, respectively). Its mean power on the sample is always kept below 1 μW (corresponding to average intensity I ~1 kW cm −2 ). The sensitivity in terms of minimum measurable absorption cross-section per unit length, ( C abs ) min , for a nanotube is a few 10 −2 nm 2 nm −1 , corresponding to relative transmission or reflection changes below 10 −4 . The SMS transmission image, |Δ T / T ( x , y )|, of a free-standing SWNT (FS-SWNT) is shown in Fig. 1b . Each individual nanotube shows up as a main central line with two satellites (in the 2 f -detection scheme) visualizing its shape. The left and right edges of the trench barely show up as vertical lines at the limits of the image. Few intense hotspots along the nanotubes reveal pollution from dust particles with sizes of the order or smaller than the light focal spot. These regions were avoided and optical measurements were performed only on ‘clean’ parts, that is, exhibiting homogeneous absorption signals along the tube ( Fig. 1c ). The R-SMS optical image, |Δ R / R ( x , y )|, of the nanotube supported by silicon substrate on one side of the trench is shown in Fig. 1d . The substrate being opaque, measurements were performed in reflection using R-SMS. Catalytic or dust nanoparticles also show up as bright spots in proximity of or away from the nanotube. Clear observation of a SWNT by either SMS or R-SMS shows the potentiality of this approach for investigating the optical properties of isolated SWNTs as a function of the incident light wavelength, polarization and environment. Absorption spectra of FS-SWNTs Many experiments demonstrated that optical transitions in CNTs arise from excitons with strong binding energy [26] , [27] , [28] even for relatively large diameters and higher-order energy transitions [10] . Each of these optical resonances is referred to as S ij or M ij , depending on the nature of the nanotube ( S for semiconducting and M for metallic) and the corresponding valence ( i ) and conduction ( j ) sub-band in the single-particle band model. Selection rules in SWNTs requires that incident light polarized parallel to the tube main axis probes transitions between sub-bands of the same index ( i = j ), and that cross-polarized light addresses transitions between sub-bands with unitary index difference (| i − j |=1) [29] , [30] . More precisely, each sub-band i shows Rydberg-like exciton states, which are composed of 4 singlet and 12 triplet states [30] . The latter are not accessible in linear optics, whereas the former are composed by one bright state at zero exciton momentum and three dark states, direct light absorption occurring only on the singlet bright state [31] , [32] . For light polarized along the tube direction, the measured spectrum of the absorption cross-section per unit length, C abs ( E ), of the FS-SWNT of Fig. 1b is plotted on Fig. 2a . Three sharp features are observed at E =1.66, 2.21 and 2.61 eV with total absorption C abs of 0.74, 0.34 and 0.38 nm 2 nm −1 , respectively, overlapping a non-resonant absorption background of amplitude ~0.14 nm 2 nm −1 . Maximum deviations on these absolute absorption measurements are ±0.025 nm 2 nm −1 , corresponding to ±0.1 × 10 −17 cm 2 per carbon atom for SWNTs diameters close to 2 nm. The same spectra are measured at different positions along the nanotube. Within the sensitivity limit of our experimental setup, no absorption is measured in the cross-polarized configuration, that is, for incident light polarized perpendicular to the nanotube main axis (open dots in Fig. 2a ). This is illustrated by plotting the absorption cross-section measured close to the resonances of lowest and highest energy as a function of the light polarization direction, relative to the CNT axis ( Fig. 2b ). This shows that the observed peaks can be ascribed to three excitonic transitions E ii between sub-bands of same index i (refs 26 , 26 , 27 , 28 , 29 , 30 , 33 ). Raman spectra measured for laser excitations close to the absorption resonances show a RBM at 128.5 cm −1 (inset of Fig. 2c ), indicating a nanotube diameter d =2.0 nm. From the diameter and energy of the absorption peaks, we infer the studied nanotube is a (22,6) semiconducting type I SWNT (defined by mod(| n − m |,3)=+1, n and m being the nanotube chiral indices) [34] , and the three resonances are identified as the S 33 , S 44 and S 55 excitonic transitions (see Supplementary Fig. S2 ). The Raman spectrum in the G-band region displays longitudinal optical and transverse optical optical phonon modes at 1,591.5 and 1,576.5 cm −1 , respectively ( Fig. 2c ), whose narrow spectral widths and frequency difference confirm a single 2 nm in diameter semiconducting nanotube is investigated [22] , [25] . Similar results were obtained for a second semiconducting type I nanotube of diameter d =1.83 nm, identified as a (14,13) SWNT ( Fig. 3 and Supplementary Fig. S3 ). In particular, the measured peak absorption cross-sections and linewidths are close to those obtained for the (22,6) SWNT ( Table 1 ). The relative variations of absorption for the different excitonic lines here are directly measured and show similar behaviour for the two CNTs, as summarized in Fig. 4a displaying the total absorption cross-sections of the suspended SWNTs, , at the investigated S ii excitonic energies. Table 1 Absorption characteristics of individual SWNTs. 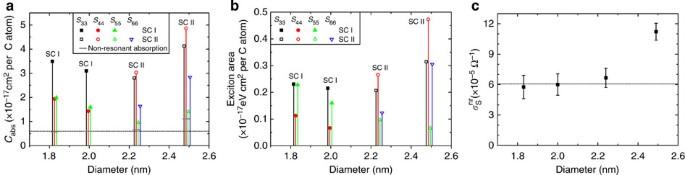Figure 4: Absorption properties of structure-assigned individual SWNTs. Quantitative absorption measurements for parallel polarization are plotted versus nanotube diameters. The SWNT family type are indicated on the figure (SC I and SC II stand for semiconducting nanotube of family type I and type II, respectively). SeeSupplementary Note 1for detailed structure assignment of each nanotube. (a) Absolute absorption cross-section at the energy transitionsSii. (b) Exciton area related to the oscillator strength of each excitonic resonance. (c) Non-resonant optical conductance. The dashed line is the ideal frequency-independent sheet conductivity of graphene. The error bars indicate the maximum uncertainty on the measured sheet conductivity. All these data are also collected inTable 1. Full size table Figure 4: Absorption properties of structure-assigned individual SWNTs. Quantitative absorption measurements for parallel polarization are plotted versus nanotube diameters. The SWNT family type are indicated on the figure (SC I and SC II stand for semiconducting nanotube of family type I and type II, respectively). See Supplementary Note 1 for detailed structure assignment of each nanotube. ( a ) Absolute absorption cross-section at the energy transitions S ii . ( b ) Exciton area related to the oscillator strength of each excitonic resonance. ( c ) Non-resonant optical conductance. The dashed line is the ideal frequency-independent sheet conductivity of graphene. The error bars indicate the maximum uncertainty on the measured sheet conductivity. All these data are also collected in Table 1 . Full size image In contrast, measurements performed on two other free-standing individual SWNTs of type II ( Supplementary Figs S4 and S5 ), with diameters determined by Raman d =2.22 and 2.52 nm, respectively, show different trends ( Table 1 and Supplementary Fig. S1 ). The individual spectra of these semiconducting SWNTs clearly present a same behaviour for the relative amplitudes of consecutive excitonic absorption cross-sections (that is, S 33 , S 44 , S 55 and S 66 ), but different as compared with the type I SWNT optical response ( Figs 2a and 3a ). For instance, the peak amplitude of the S 44 resonance is weaker than the S 33 one in type I semiconductor SWNTs (with similar spectral widths) but is slightly increased for type II SWNTs (the ratio of the total absorption cross-section per unit length being smaller than 0.5 and slightly larger than 1 for the type I and II SWNTs, respectively, Fig. 4a ). Such a behaviour is first observed here with a direct absorption measurement and is consistent with theoretical predictions for resonant Raman intensities [35] . To more precisely analyse the SWNT absorption spectrum at the excitonic peaks, including linewidth and background effects, the excitonic transitions were fitted with Voigt profiles. These take into account convolution of the excitonic line, assumed to exhibit a Lorentzian shape, with the Gaussian spectral profile of the incident light beam. Adding a uniform non-resonant absorption background, a good reproduction of the measured spectrum is obtained (dashed lines in Figs 2a and 3a and Supplementary Fig. S1a,d , the small spectral features not reproduced being commented later). The extracted spectral FWHM and absorption resonance integrated area (or equivalently, peak excitonic absorption ) are reported in Table 1 for the excitonic resonances of investigated type I and II SWNTs. The exciton peak linewidths generally tends to increase with transition energy, for instance from about 50 meV for the S 33 and S 44 resonances of the type I SWNTs to about 100 meV for the S 55 one. These values measured here directly from the absorption spectra are consistent with those generally reported in individual suspended nanotube Rayleigh or Raman studies [10] , [11] , [13] . The integrated spectral area of the excitonic line is proportional to the exciton oscillator strength and is thus characteristic of the absorption strength, independently of the spectral width. It thus permits to precisely analyse the dependence of the oscillator strength on the excitonic transition and nanotube structure. It exhibits a non-monotonic variation with an ‘oscillating’ type of behaviour, as it increases then decreases for two adjacent lines in both type I and type II semiconducting SWNTs ( Fig. 4b ). However, for the type I family, the oscillator strength first decreases from the S 33 to the S 44 transitions, increasing again to the S 55 one, whereas for the type II family an opposite variation is measured from the S 33 to the S 66 transitions. Our experimental determination of the relative oscillator strength variations as a function of the transitions is in agreement with recent theoretical predictions [36] . In particular, the computed dependencies on the nanotube structure (family type and chiral angle) are consistent with our results. The sensitivity of SMS experimental method also allows observation of additional small spectral features, as in the parallel absorption spectrum of the (14,13) SWNT ( Fig. 3a ). The two broad structures about 200 meV above the S 33 and S 44 transitions are ascribed to the bright K-momentum phonon sideband (PSB) of the corresponding S ii dark excitons [27] , [37] , [38] , [39] . They were included in the fit using an asymmetric sideband lineshape introducing a broadening of about 50 meV (refs 38 , 39 ). In fact, the PSB of the S 33 transition for the (22,6) SWNT can also be identified around 1.86 eV ( Fig. 2a ), but overlaps other features between 1.9 and 2.05 eV as discussed below. The weaker PSB-related absorption in the (22,6) than (14,13) SWNT suggests chirality-dependent coupling (chiral angles ~12° and ~29° for the (22,6) and (14,13) SWNT, respectively) between K-momentum dark excitons and near zone-edge optical phonons, as discussed for photoluminescence excitation spectroscopy [39] . The three sharper side peaks below the S 33 transition of the (14,13) SWNT are equally spaced by about 130 meV ( Fig. 3a ), close to zone-edge transverse acoustic phonon energy, which could reflect phonon-assisted absorption. However, their absorption (at 1.68 eV, see Fig. 3a open dots) is less polarization dependent, possibly suggesting the presence of a crossed optical transition S ij , as in recent polarized photoluminescence excitation experiments [27] . More generally, other possible physical origins for side features in CNT optical response could originate from excited excitonic states within each sub-band transition S ii (refs 32 , 40 ). Further temperature- and polarization-dependent investigations, as well as lineshape analysis, would help to determine the mechanisms at the origin of all these absorption features. Substrate effects on the optical response As our optical approach permits to investigate single nanotubes either suspended or on an opaque substrate (using either SMS or R-SMS), it offers the unique possibility of measuring quantitative modifications of the optical response of the same SWNT in these two situations. The absorption spectrum measured by R-SMS on the SiO 2 /Si-supported part of the (14,13) SWNT (SI-SWNT) shows large modifications as compared with that measured by SMS on its FS-SWNT part ( Fig. 3a,d ). For light polarized parallel to the tube axis, the three excitonic peaks S 33 , S 44 and S 55 are still visible but are red-shifted and considerably broadened, and their relative peak amplitude modified, as compared with the FS-SWNT case. These effects can be quantified by fitting the measured SI-SWNT spectrum ( Fig. 3d dashed line), yielding a red shift of 60 meV and a five times broadening of the S 33 and S 44 resonances ( Table 1 , third row). The S 55 transition is less altered, as it is red-shifted by 20 meV and its linewidth increasing by less than a factor of three (the S 33 , S 44 and S 55 exhibiting similar width). The measured red shifts and broadening are in agreement with photoluminescence or Raman excitation spectroscopy on supported SWNT as compared with suspended ones, and have been mainly ascribed to substrate-induced dielectric screening and exciton localization at defect sites [13] . As SMS and R-SMS provide the absolute absorption spectra, the impact of the substrate effects on the background and excitonic peak absorption cross-sections can be analysed. The non-resonant absorption remains close to its value for the FS-SWNT, ~0.14 nm 2 nm −1 (that is, 0.6 × 10 −17 cm 2 per carbon atom, Table 1 ). The peak values of the absorption cross-section at the excitonic resonances are differently modified ( Table 1 ). For instance, the S 44 transition becomes stronger than the S 33 and S 55 , their width staying comparable, suggesting different coupling with the substrate (note, however, that the S 55 transition is at the limit of our SMS setup tunability due to the microscope objective transmission, and its amplitude may also be affected by Fabry–Perot corrections due to the substrate structure, see Methods). These measurements over a large spectral range also make possible analysis of the evolution of the oscillator strength of the excitonic transitions due to deposition, the line areas for the SI-SWNT showing an increase of the oscillator strength as compared with the FS-SWNT for the different transitions. Interestingly, the absorption cross-section measured here on a (14,13) semiconducting SWNT is in very good agreement with the first R-SMS measurement performed for few wavelengths on the chirality-identified (18,5) type I SWNT, of diameter d =1.65 nm and grown by CVD on 300 nm silica on silicon substrate [15] . In particular, the reported out-of-resonance absorption, ~0.6 × 10 −17 cm 2 per carbon atom, is very close to that measured here, and the S 33 excitonic absorption per carbon atom of the (18,5) SWNT ( ~1.2 × 10 −17 cm 2 per carbon atom, after subtraction of ) is consistent with that obtained here on the (14,13) SI-SWNT for the same transition ( ~1 × 10 −17 cm 2 per carbon atom). An additional striking feature is the large reduction of light polarization effect. Significant absorption is still observed for the supported section of the tube for light polarized perpendicularly to the tube axis (see open dots in Fig. 3d ), with, however, only weak remaining structures (except in the S 55 spectral region). Although the absorption is almost fully polarized in the free-standing region, the SI-SWNT spectra exhibit a photon energy-dependent contrast factor between light polarized parallel ( ) or orthogonal ( ) to the nanotube axis ranging from 2:1 to 4:1 ( Fig. 3b,e , where the polarization-dependent data are fitted by , θ =0 being the direction parallel to the nanotube axis). Weakening of the polarization contrast can be ascribed to softening of the antenna effect for deposited CNTs, associated with weakening of the depolarization field inside the tube [12] , [15] . Moreover, its wavelength dependence suggests different interaction induced by nanotube–substrate coupling and possible contribution from crossed-polarized S ij transitions. The impact of the substrate has been confirmed by Raman measurements. Although no significant change is observed for the RBM frequency and width ( ω RBM =139 and 138 cm −1 , with a FWHM of 11 and 13 cm −1 for the FS-SWNT and SI-SWNT, respectively), both the longitudinal optical and transverse optical modes of the G-band are upshifted and broadened in the SI-SWNT, with apparition of additional peaks associated with modes of other symmetries ( Fig. 3f ) [13] . Possible contributions for these environment-induced Raman and absorption spectral modifications have been mainly ascribed to dielectric, chemical and mechanical effects [41] , [42] , [43] , [44] , [45] . From a general point of view, the absorption cross-section of a nano-object is related to the imaginary part of its polarizability (or, equivalently, to the real part of its optical conductivity) and is possibly affected by local field effects [46] . For an elongated nanotube of diameter d and length L , with d << λ << L , in a homogeneous medium of refractive index n m , the local field is actually identical to the incident electric field when light is polarized parallel to the nanotube axis. In this configuration, the absorption cross-section per unit length, C abs, L , computed in the quasi-static approximation then simply writes: C abs, L = πdZσ S , where Z =( ε 0 cn m ) −1 is the impedance of the medium and σ S is the real part of the nanotube sheet conductivity. The absorption cross-section per carbon atom is then given by: C abs,C = C abs, L d −1 = π Zσ S , where a C is the radius of the equivalent surface occupied by a carbon atom in the crystalline lattice. Using this simple model, the absolute absorption spectra of SWNTs measured here yield access to their optical conductance σ S ( ω ) at the excitonic transitions or out of resonance. The three smallest semiconducting SWNTs investigated in this work with diameter d in the 1.8–2.2 nm range show a non-resonant absorption cross-section =(0.6±0.1) × 10 −17 cm 2 per carbon atom ( Table 1 ). This value is almost independent of the nature of the nanotube (type I or II) and is not affected by the presence of a substrate, suggesting it reflects an intrinsic property of SWNT (at least for small SWNTs, only the largest-diameter nanotube with d =2.5 nm showing a larger non-resonant absorption, see Table 1 —however, in this CNT the orthogonally polarized absorption is also larger than the one measured for smaller tubes, see Supplementary Fig. S1d ). Using this value and the previous expression with n m =1 for FS-SWNT, a non-resonant optical conductance is deduced =(6±1) × 10 −5 Ω −1 ( Fig. 4c ). This value is close to the frequency-independent ideal sheet conductivity of graphene, = σ g = G 0 π /2, where G 0 = e 2 / h ≈3.9 × 10 −5 Ω −1 is the quantum of conductance [47] , [48] , [49] . In contrast to the energy-dependent optical absorption of graphene [48] , here remains comparable to the ideal (that is, related to the fine structure constant α = e 2 /(4 π ε 0 ħc )) graphene absorbance, A = C abs,C / π = πα , in the 1.5–3.0 eV spectral range, suggesting different influences of interband transitions on CNT absorption [50] . Similarly, the absorption cross-sections per unit length measured for the excitonic transitions can be expressed in terms of optical conductances σ S ( ω ). For the investigated SWNT, they are found to be a few units of quantum conductance G 0 , σ S ( ω ) varying in the 4 G 0 –9 G 0 range for the S 33 and S 44 transitions (see also Table 1 ). This range is compatible with the results of recent Rayleigh scattering experiments [14] . However, much larger systematic dependence of σ S ( ω ) (or of ) on the excitonic transitions, and thus of the associated oscillator strength, is demonstrated by our absorption measurements ( Fig. 4a,b ). In conclusion, the absolute absorption spectra of individual free-standing or deposited semiconducting SWNTs were measured by SMS in a broad optical range. Quantitative determination of their optical absorption spectra permits determination of their absorption cross-section per unit length and associated resonance oscillator strength at the excitonic transitions. Systematic trend of the latter is demonstrated with an oscillatory kind of behaviour for adjacent excitonic lines, having opposite variations in type I and II semiconducting SWNTs. A significant non-resonant absorption background is observed in all investigated SWNT, either free-standing or supported, with an amplitude comparable to the ideal graphene absorbance. Comparison of the spectra measured for the same SWNT free-standing or deposited on a SiO 2 /Si substrate directly shows that SWNT interaction with a substrate induces a large broadening of the excitonic transitions concomitant with a shift of their frequency, and an increase of their oscillator strength together with a strong depolarization effect. The quantitative results reported here are of particular relevance for investigation and modelling of the intrinsic electronic properties of CNTs either free-standing or supported (a situation relevant for practical applications). Furthermore, the experimental approach developed here open many possibilities for investigating other individual nanotubes, as metallic ones, or to the impact of nanotube interaction in bundles. Spatial modulation spectroscopy SMS is a far-field microscopy technique based on tightly focusing a light beam on a nano-object whose position is modulated. For displacement along the y direction by Δ y 0 , the object is located at ( x 0 , y 0 +Δ y 0 ). This reflects in modulation of the transmitted power Δ P T ≈−Σ ext { I ( x 0 , y 0 +Δ y 0 )− I ( x 0 , y 0 )}, where I ( x , y ) is the incident light-beam intensity profile in the focal plane. It is directly proportional to the nano-object extinction cross-section Σ ext , that can be identified to the absorption cross-section Σ abs for small absorbing nano-objects as SWNT (the scattering cross-section being negligible as compared with the absorption one). For harmonic modulation of the particle position at frequency f (≈1.5 kHz), high-sensitivity synchronous detection at frequency f or 2 f of Δ P T is performed [18] , [51] . The optimal amplitude of modulation is close to the FWHM, d FWHM , of the focused laser beam [52] . For elongated nano-objects as CNTs, the absorbed power is obtained by integrating C abs I ( x , y ) ds over the probed nanotube zone, where s is the curvilinear abscissa along the one-dimensional object of length L and C abs is its absorption cross-section per unit length. The amplitude of the relative transmission change, Δ T / T =Δ P T / P T , is then set by C abs , that can thus be quantitatively determined. The best signal contrast is obtained for a modulation direction perpendicular to the nanotube axes and more precise nanotube localization achieved for 2 f signal demodulation [15] . In this configuration, SMS images obtained by scanning the sample position ( x 0 , y 0 ) display CNTs as triple-line peaks that follow the morphology of the nanotube (see Fig. 1 ). FS-SWNTs suspended over a trench were imaged using SMS in the above described transmission configuration. Their extremities, deposited on a silicon substrate covered by a 100-nm silica layer, were investigated using a variant of the SMS technique in reflection configuration (R-SMS) adapted to opaque substrates [15] . Absorption spectra and polarization optical responses were obtained by measuring C abs at different wavelengths and for different incident light polarization ( Figs 2 and 3 and Supplementary Fig. S1 ). In the R-SMS configuration, Fabry–Perot effects associated with the presence of a layered substrate have to be taken into account for extracting the absorption cross-section from reflectivity measurements. First-order corrections of these effects have been used [15] , as in the broadband spectrum of Fig. 3d . These are strictly valid close to the Fabry–Perot maxima (that is, around 2.1 eV for the used substrates, close to the S 33 and S 44 transitions displayed in Fig. 3d ), but may affect the actual amplitude of the optical response at other wavelengths (in particular, around the S 55 transition). Raman spectroscopy Resonant Raman scattering measurements were carried out using an iHR550 Jobin-Yvon spectrometer (gratings 1,800 or 1,200 grooves per mm, precision ≈±1 cm −1 ) equipped with a liquid-nitrogen-cooled, back-illuminated silicon charge-coupled device detector in a micro Raman backscattering configuration. The home-made microscope is equipped with a × 100 objective (numerical aperture=0.9). The samples were mounted on a three-axis piezoelectric stage (PIMars P-563 PI) to ensure the precise positioning and focusing of the laser spot. Incident excitations from various continuous wave lasers were used: HeNe at 632.8 nm (1.96 eV), diode-pumped solid-state lasers at 457 nm (2.71 eV), 532 nm (2.33 eV) and 561 nm (2.21 eV), and a Ti-Sapphire filtered using a tunable laser line filter [53] in the near infrared. In all the measurements, the incident light polarization is along the nanotube axis. To avoid heating effects, the laser intensity impinging the sample was kept below 100 kW cm −2 . CNT sample fabrication The suspended nanotubes were synthesized by CVD on home-made silica on silicon slit substrates using the method previously reported [54] , [55] , [56] . The catalyst consists of 5 Å Fe thin films deposited by thermal evaporation on SiO 2 /Si substrates. During the CVD, the catalyst substrates were put side by side with the slit substrates. The substrates were oriented with the catalyst side towards the gas inlet. The sample held in a quartz tube was kept outside the heated zone during temperature ramping of the furnace. Before heating, all gas lines and the reactor tube were purged by argon at a flow rate of 800 sccm for 30 min. Next, the furnace was heated to 950 °C or 1,000 °C at a ramping rate of 20 °C min −1 . To carry ethanol to the furnace, Ar at a flow of 10 or 15 sccm was passed through a bubbler containing ethanol (kept at room temperature ~25 °C). When the temperature reached the synthesis temperature, argon was replaced by hydrogen and ethanol/argon at flow rates (1:1 ratio) of 10 or 15 sccm. After 5 min, the furnace was slid to the sample position to fast heat the sample and to grow CNTs. The synthesis durations were 30 min. After that, hydrogen and ethanol vapour were replaced by pure Ar at a flow rate of 30 sccm, the furnace was switched off and was slid to the initial position to fast cool the samples. How to cite this article: Blancon, J. -C. et al. Direct measurement of the absolute absorption spectrum of individual semiconducting single-wall carbon nanotubes. Nat. Commun. 4:2542 doi: 10.1038/ncomms3542 (2013).